Visualization of a ferromagnetic metallic edge state in manganite strips Recently, broken symmetry effect induced edge states in two-dimensional electronic systems have attracted great attention. However, whether edge states may exist in strongly correlated oxides is not yet known. In this work, using perovskite manganites as prototype systems, we demonstrate that edge states do exist in strongly correlated oxides. Distinct appearance of ferromagnetic metallic phase is observed along the edge of manganite strips by magnetic force microscopy. The edge states have strong influence on the transport properties of the strips, leading to higher metal–insulator transition temperatures and lower resistivity in narrower strips. Model calculations show that the edge states are associated with the broken symmetry effect of the antiferromagnetic charge-ordered states in manganites. Besides providing a new understanding of the broken symmetry effect in complex oxides, our discoveries indicate that novel edge state physics may exist in strongly correlated oxides beyond the current two-dimensional electronic systems. Edge states emerging at the symmetry breaking boundaries are not only highly intriguing from fundamental physics point of view but also very promising for next-generation electronic devices, which have been already studied intensely in topological insulators [1] , [2] and graphene ribbons [3] , [4] , [5] . However, to date, there have been no reports on the existence of edge states in strongly correlated oxides. The colossal magnetoresistive (CMR) manganites belong to a classical strongly correlated oxides system. Owing to a strong correlation between lattice, spin, charge and orbital, competing electronic states in manganites often have close energy scales leading to rich phase diagrams and spatial coexistence of different electronic phases known as electronic phase separation (EPS), which makes the properties of manganites very sensitive to any external fields. EPS has a strong influence on colossal magnetoresistance and metal–insulator transitions (MIT) in manganites [6] , and the effect becomes even more pronounced when manganites are fabricated into strips [7] , [8] , [9] , [10] . These features make manganites the ideal system in which to study edge state physics among complex oxides systems. Although surface [11] , [12] , [13] and grain boundary effects [14] , [15] , [16] , [17] have been observed in manganites systems, it is very interesting to verify whether broken symmetry effect can introduce intrinsic edge states in manganites, especially when EPS dominates the system. For this reason, we have chosen a model system of La 0.325 Pr 0.3 Ca 0.375 MnO 3 (LPCMO) which has been well known for its striking large length scale EPS between ferromagnetic metallic (FM) and CE-type antiferromagnetic charge-ordered insulating (CE) phases [18] . In this work, we show that FM edge states do exist in manganite strips. Our observation is made by using magnetic force microscopy (MFM) and transport measurement techniques to study manganite strips as a function of temperature and magnetic field. The edge states are robust in the sense that they exist independent of substrate strain, cycles of temperature and magnetic field change, and the history in ambient atmosphere. The critical temperature for the edge states is observed to be considerably higher than that of the FM phase in regions away from the edge. Monte Carlo simulations based on the two-orbital double-exchange model show that the physical origin of the edge states is associated with the broken symmetry effect of the antiferromagnetic charge-ordered states in manganites. Magnetic properties and MFM imaging LPCMO strips are fabricated from epitaxial thin films grown on SrTiO 3 (100) substrates by optical lithography. 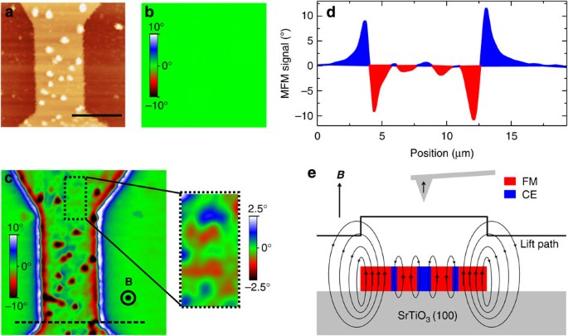Figure 1: The geometry and magnetic structures of LPCMO strip on SrTiO3(100). (a) Atomic force microscopy and (b) MFM images of the 10-μm LPCMO strip at 300 K under zero field. (c) The MFM image of the 10-μm LPCMO strip at 120 K under magnetic field (B=9 T, pointing out of the sample surface) and the zoom-in of the dotted areas (3 μm × 6 μm) with a scale of 5°. Scanned areas in (a–c) are 25 μm × 25 μm. The black scale bar inais 10 μm. (d) Line profile of the dashed black line inc. (e) Its corresponding schematic of the magnetic structures during the MFM imaging process. Ind, negative signals in red stand for the attractive force between the sample and tip (thus FM state), whereas positive signals in blue stand for the repulsive force (thus, CE state). Ine, FM states are labelled in red, whereas CE states are shown in blue. The black arrows show the magnetic moment directions of the tip and the sample under the magnetic fieldB. The black lines show the lift path of the tip and the black circles show the magnetic flux of the sample. The strip shows clear ferromagnetic edge phases at the sample boundaries. Figure 1a,b shows the topography and the magnetic image of a 10-μm-wide strip (80 nm in thickness) acquired by atomic force microscopy and MFM under zero magnetic field at 300 K. The MFM image shows no contrast since the Curie temperature ( T c) of LPCMO is well below 300 K (~210 K for the 80-nm parent film). Figure 1: The geometry and magnetic structures of LPCMO strip on SrTiO 3 (100). ( a ) Atomic force microscopy and ( b ) MFM images of the 10-μm LPCMO strip at 300 K under zero field. ( c ) The MFM image of the 10-μm LPCMO strip at 120 K under magnetic field ( B =9 T, pointing out of the sample surface) and the zoom-in of the dotted areas (3 μm × 6 μm) with a scale of 5°. Scanned areas in ( a – c ) are 25 μm × 25 μm. The black scale bar in a is 10 μm. ( d ) Line profile of the dashed black line in c . ( e ) Its corresponding schematic of the magnetic structures during the MFM imaging process. In d , negative signals in red stand for the attractive force between the sample and tip (thus FM state), whereas positive signals in blue stand for the repulsive force (thus, CE state). In e , FM states are labelled in red, whereas CE states are shown in blue. The black arrows show the magnetic moment directions of the tip and the sample under the magnetic field B . The black lines show the lift path of the tip and the black circles show the magnetic flux of the sample. The strip shows clear ferromagnetic edge phases at the sample boundaries. Full size image With decreasing temperature, magnetic contrast becomes increasingly apparent in the 10-μm strip. Figure 1c shows a MFM image of the strip acquired at 120 K under a 9-T field applied normal to the substrate surface. The field is high enough to drive the magnetization of both the sample and the tip to align along the field direction. Pronounced ferromagnetic edge phases can be clearly seen along both edges of the strip. Inside the strip, the usual micron-scale EPS domains still exist, as shown in the magnified area of the strip outlined by the black box in Fig. 1c . The marked line profile across the strip and its corresponding schematic of the magnetic structures are shown in Fig. 1d,e , which indicates that the ferromagnetic signal of the edge phases is ~10 times larger than that of the EPS inside the strip ( Supplementary Note 1 and Supplementary Fig. 1 ). The spotty strong MFM signals inside the strip are caused by droplets (formed during thin film growth) rather than any intrinsic mechanisms (one-to-one correspondence between droplets and strong magnetic signals in Fig. 1a,c is observed). We note that changing the scanning direction by 90° does not affect the appearance of the edge phases, which rules out the possibility that the edge phases are caused by scanning effect or any other external noises ( Supplementary Fig. 2 ). In addition, electrostatic force microscopy measurements show little contrast at the strip edge ( Supplementary Fig. 3 ); the MFM contrast is reversed when switching the magnetization direction of the tip ( Supplementary Fig. 4 ). The hysteresis behaviour and the non-zero remanence of the MFM signal at 10 K further demonstrate that the edge phases are ferromagnetic ( Supplementary Fig. 5 ). These additional experimental data all indicate that the MFM contrast is from magnetic origin ( Supplementary Note 2 ). We also note that the signal of the FM edge phase in the same sample does not change even after more than a year of placement in the ambient atmosphere. The dependence of the edge phases on temperature and strip width is shown in Fig. 2 . For the 10-μm strip, with decreasing temperature, the magnetic signal of the edge phases increases in both amplitude and lateral size, and remains clearly distinguishable from that of the EPS domains inside the strips. For the 3-μm strip, the edge phases, while distinguishable from the interior EPS domains at 200 K, expand their lateral dimension and merge together to fill the strip at low temperatures. This is even more obvious for the 1.5-μm strip. The two edge phases percolate and fill the strips even at 300 K, which is well above the Curie temperature of the parent film. The merging of the edge phases leads to a strong enhancement of ferromagnetism in narrow strips as compared with that of the films ( Supplementary Fig. 6 ). 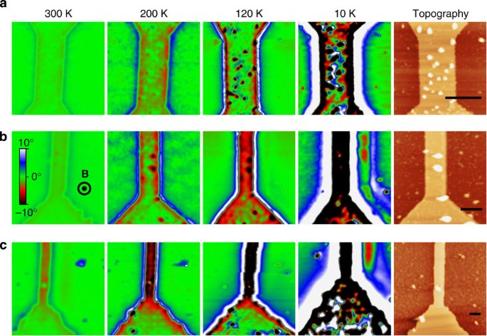Figure 2: Strip width and temperature dependence of LPCMO edge phases. The MFM images of LPCMO under 9 T field (Bis pointing out of the sample surface) with (a) 10, (b) 3 and (c) 1.5 μm strips, followed by their topography images, Scanned areas are 20 μm × 20 μm ina, and 15 μm × 15 μm inb,c. The black scale bars are 10 μm ina, 3 μm inband 1.5 μm inc. In narrow strips, the edge phases show great enhancement of magnetic signals and give much higher Curie temperatures. Figure 2: Strip width and temperature dependence of LPCMO edge phases. The MFM images of LPCMO under 9 T field ( B is pointing out of the sample surface) with ( a ) 10, ( b ) 3 and ( c ) 1.5 μm strips, followed by their topography images, Scanned areas are 20 μm × 20 μm in a , and 15 μm × 15 μm in b , c . The black scale bars are 10 μm in a , 3 μm in b and 1.5 μm in c . In narrow strips, the edge phases show great enhancement of magnetic signals and give much higher Curie temperatures. 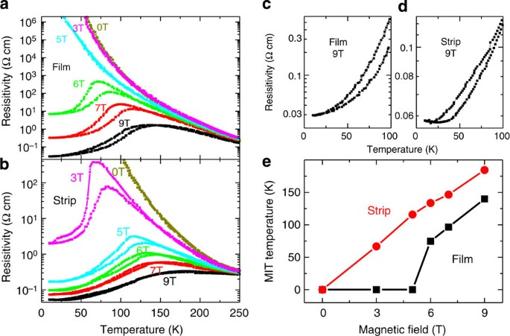Figure 3: The transport properties of LPCMO. The transport data of (a) the LPCMO film and (b) the 1.5-μm strip under magnetic fields of 0 T (dark yellow), 3 T (magenta), 5 T (cyan), 6 T (green), 7 T (red) and 9 T (black). (c,d) Magnification of the film and 1.5 μm strip transport data under 9 T at low temperatures. (e) The comparison of metal–insulator transition (MIT) temperatures between the film (black squares) and the 1.5-μm strip (red dots) derived from the cooling curve ina,b. The narrow strip exhibits higher MIT temperatures and lower resistivity than its parent film, which indicates that the edge phases are metallic. Full size image Transport properties Figure 3 shows comparison of transport properties of the parent film ( Fig. 3a ) and the 1.5-μm strip ( Fig. 3b ). Surprisingly, the strip shows considerably lower resistivity and much higher MIT temperatures compared with those of the film when the magnetic field is <7 T. Remarkably, the low-temperature resistivity of the strip is >6 orders of magnitude lower than that of the film at 3 and 5 T. This strongly suggests that the edge phases of the strip are not only ferromagnetic but also metallic. At even higher magnetic field (>7 T), the CE phase in the film is completely melted by the magnetic field and the whole film becomes metallic. This explains why the resistivity of the film becomes smaller than that of the strip in the metallic state at 9 T ( Fig. 3c,d ). However, even at 9 T field, the strip still has a considerably higher MIT temperature than the film, which is consistent with our MFM observations in Fig. 2 . The comparison of the field-dependent MIT temperatures of the strip and the film is summarized in Fig. 3e . Figure 3: The transport properties of LPCMO. The transport data of ( a ) the LPCMO film and ( b ) the 1.5-μm strip under magnetic fields of 0 T (dark yellow), 3 T (magenta), 5 T (cyan), 6 T (green), 7 T (red) and 9 T (black). ( c , d ) Magnification of the film and 1.5 μm strip transport data under 9 T at low temperatures. ( e ) The comparison of metal–insulator transition (MIT) temperatures between the film (black squares) and the 1.5-μm strip (red dots) derived from the cooling curve in a , b . The narrow strip exhibits higher MIT temperatures and lower resistivity than its parent film, which indicates that the edge phases are metallic. Full size image Physical origin of edge phases and theoretical simulation We now discuss the physical origin of the edge phases. The edge-damaging effect caused by wet etching when fabricating the strips can be ruled out since such kind of structural damages will always drive manganite systems less ferromagnetic, especially when the Ca doping of LPCMO is optimized at 3/8 (ref. 19 ) We have also used time-of-flight secondary ion mass spectrometry technique (TOF-SIMS) to check the La/Pr ratio across the strips, which reveals no difference between the edge and the center of the strips ( Supplementary Fig. 7 ). Strain relaxation at the strip edge can be another possible cause for the observed edge phase, since the MIT temperature of LPCMO films is found very sensitive to the lattice mismatch of substrates [20] . When grown on the present SrTiO 3 (100) substrate, the LPCMO strips are under tensile strain (+1.6%). To verify the strain effects, we have performed additional experiments on LPCMO strips grown on SrLaGaO 4 (100) (no strain) and LaAlO 3 (100) (compressive strain, −1.4%) substrates. As shown in Supplementary Figs 8 and 9 , pronounced edge phases have been consistently observed in these two systems as well, which strongly indicates that the observed edge phase is not caused by the edge strain effect. This means that the edge phase is clearly different from the strain-induced grain boundary effect observed in manganites bi-crystals [14] , [15] or polycrystals [16] , [17] . A plausible mechanism of the edge phases in the manganite strips is the broken symmetry effect of the CE phase. To verify this, we used the standard two-orbital double-exchange model in the half doping system, whose CE-type spin structures are believed to be most stable [21] (see Supplementary Notes 3 and 4 for details). The superexchange ( J AF ) has been included while the Jahn–Teller distortion is neglected for simplicity and clarity. First, we compared the energy of FM state and CE state as a function of J AF as shown in Fig. 4a . Next, two CE ground state points with J AF =0.12 (close to the phase transition point thus fragile) and 0.14 (robust) were selected to calculate the edge effect. A low-temperature Monte Carlo simulation is used on a two-dimensional 16 × 8 lattice with full-periodic boundary conditions to simulate the bulk without edges, while half-periodic/open boundary conditions are used to simulate the effect of two edges. As a result, the spin structures with full-periodic boundary conditions at these two points exhibit a perfect CE pattern with zig-zag chains running through the whole lattice ( Fig. 4b,d ), while the edges indeed break the CE-type zig-zag pattern with a FM tendency and form ferromagnetic edge states within a few unit cells ( Fig. 4c,e ). Although the Ca doping ratio in our experimental system case is 3/8, it has been observed that this kind of CE-type state still exists [22] , [23] . The only difference is that the CE-type state in 3/8 Ca-doping system is weaker and easier to be disturbed owing to the doping offset to its optimized half doping, which will benefit the emergence of ferromagnetic edge states. 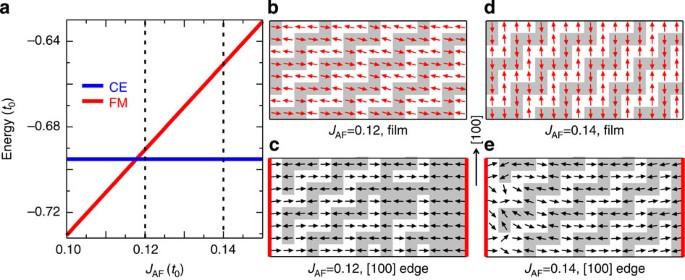Figure 4: Physical origin of the edge phases. (a) Ground state calculation using the standard two-orbital double-exchange model on two-dimensional lattice. The energies of FM state (red curve) and CE state (blue curve) are plotted as a function of superexchangeJAF. All energies are in unit oft0(the double-exchange hopping). Simulated spin structure on 16 × 8 lattice at the fragile CE state (JAF=0.12) with (b) full-periodic boundary conditions (shown by short red arrows) and (c) two [100] cutting edges(shown by short black arrows). Simulated spin structure on 16 × 8 lattice at the robust CE state (JAF=0.14) with (d) full-periodic boundary conditions (shown by short red arrows) and (e) two [100] cutting edges(shown by short black arrows). Inc,e, the long direction is cut with two edges (marked as red bold lines), whereas the short direction is periodic connected without edges. The long black arrow indicates [100] direction of the system. The edges show obvious ferromagnetic tendency. Figure 4: Physical origin of the edge phases. ( a ) Ground state calculation using the standard two-orbital double-exchange model on two-dimensional lattice. The energies of FM state (red curve) and CE state (blue curve) are plotted as a function of superexchange J AF . All energies are in unit of t 0 (the double-exchange hopping). Simulated spin structure on 16 × 8 lattice at the fragile CE state ( J AF =0.12) with ( b ) full-periodic boundary conditions (shown by short red arrows) and ( c ) two [100] cutting edges(shown by short black arrows). Simulated spin structure on 16 × 8 lattice at the robust CE state ( J AF =0.14) with ( d ) full-periodic boundary conditions (shown by short red arrows) and ( e ) two [100] cutting edges(shown by short black arrows). In c , e , the long direction is cut with two edges (marked as red bold lines), whereas the short direction is periodic connected without edges. The long black arrow indicates [100] direction of the system. The edges show obvious ferromagnetic tendency. Full size image The simulation shows strong evidence that the large-scale edge phases we observed come from the broken symmetry effect induced edge states in LPCMO. The CE-type phase has the tendency to form ferromagnetic edge states by principle. However, since the electronic states in the phase-separated conditions are very sensitive to the environment, these nanoscale edge states could have as a seed and trigger even larger scale edge phases in the real mesoscopic strip. This kind of seeding effect on LPCMO surface has been observed through surface exchange coupling with ferromagnetic iron nanodots [24] . Moreover, the width of edge phases at initial stage acquired by MFM is ~1 μm, which is the typical length scale of EPS domains in LPCMO. Therefore, we can claim that these observations are the intrinsic FM edge states of LPCMO. In summary, we have discovered pronounced FM edge state in manganite strips by MFM and transport measurements. The edge states could provide us a new way (by size or geometry) to control the electronic phase separation in manganites, and thus their physical properties without using external fields and chemical doping. The fact that the edge state has a higher critical temperature is useful to increase the Curie temperature of manganites strips, which is highly desirable for device applications of the CMR manganites materials. Moreover, our observation indicates that robust edge state does exist in strongly correlated oxides systems, which opens the door to study edge state physics and to discover novel phenomena in these already interesting systems. Sample preparation LPCMO thin films were grown on single crystal SrTiO 3 (100), LaAlO 3 (100) and SrLaGaO 4 (100) substrates by laser (248 nm, 1 J cm −2 fluence, 2 Hz) molecular beam epitaxy at 820 °C in a flowing oxygen (10% ozone) environment under a pressure of 3 mTorr and post annealed at 950 °C for 3 h in the oven after growth. Film quality was confirmed by atomic force microscopy and X-ray diffraction. Device fabrication The LPCMO strips were fabricated by the conventional optical lithography and KI:HCl:H 2 O (1:1:1) wet etching. Au electrodes with Cr buffer layers were evaporated and patterned on the samples for transport measurements by electron beam lithography and lift-off technique. MFM and transport measurements MFM images and the transport measurements were carried out in Physical Property Measurement System with scanning probe microscope (Quantum Design). Commercial Co/Cr-coated and home-made Co/Pt high coercivity [25] MFM probes were used in the MFM dual-pass mode with a lift height of 100 nm (step height of the strip is 80 nm) in order to remove the morphology contribution from MFM signals. TOF-SIMS TOF-SIMS 5–100 system with Bi-LMIG source (30 KeV) was utilized to carry out the distribution of La and Pr on the LPCMO strip, by summing up all the La and Pr relevant ions’ signals, respectively. The distribution results of Ca and Mn are also uniform, while the signals of K, I and Cl are under the detection limits (noise level). How to cite this article: Du, K. et al . Visualization of a ferromagnetic metallic edge state in manganite strips. Nat. Commun. 6:6179 doi: 10.1038/ncomms7179 (2015).